Spatial separation of photogenerated electrons and holes among {010} and {110} crystal facets of BiVO4 Charge separation is crucial for increasing the activity of semiconductor-based photocatalysts, especially in water splitting reactions. Here we show, using monoclinic bismuth vanadate crystal as a model photocatalyst, that efficient charge separation can be achieved on different crystal facets, as evidenced by the reduction reaction with photogenerated electrons and oxidation reaction with photogenerated holes, which take place separately on the {010} and {110} facets under photo-irradiation. Based on this finding, the reduction and oxidation cocatalysts are selectively deposited on the {010} and {110} facets respectively, resulting in much higher activity in both photocatalytic and photoelectrocatalytic water oxidation reactions, compared with the photocatalyst with randomly distributed cocatalysts. These results show that the photogenrated electrons and holes can be separated between the different facets of semiconductor crystals. This finding may be useful in semiconductor physics and chemistry to construct highly efficient solar energy conversion systems. Charge separation has a key role in determining solar energy conversion efficiency of semiconductor-based systems for producing solar electricity and solar fuels through solar cells [1] , [2] , [3] , [4] , photoelectrocatalysis [5] , [6] , [7] , [8] and photocatalysis [9] , [10] , [11] , [12] , [13] . As a key step in energy conversion, electron-hole pairs generated by light absorption need to be separated and transferred to the surface of the semiconductors [1] , [9] , [14] , [15] , [16] , [17] . Hence, an in-depth understanding of charge separation within semiconductors is desirable for the construction of an efficient solar energy conversion system. Recent investigations on crystal facet engineering of semiconductors have demonstrated that photoexcited electrons and holes may be driven to different crystal facets. Thus, certain facets of a semiconductor prefer reduction while others favour oxidation [18] , [19] , [20] . However, reports on the reduction and oxidation reaction facets on the same semiconductor crystal (such as TiO 2 ) were often contradictory in the literature [21] , [22] , [23] , [24] , [25] , [26] . For example, it was reported that rutile {011} and anatase {001} faces provided the sites for oxidation, while the rutile {110} and anatase {101} faces offered the sites for reduction [24] . Similar phenomena were also reported in other references [27] , [28] , [29] . However, some references observed higher photocatalytic oxidation activity of organics on anatase nanocrystals with well-faceted {101} surfaces than that of the above-mentioned {001} facet [30] , [31] , [32] . Farneth et al . [21] concluded that the fine Ag particles are mostly deposited by reduction of Ag + on the {110} face of TiO 2 , while Hotsenpiller et al . [22] reached the conclusion that the Ag particles were photocatalytically deposited at higher velocities on the {001} and {011} facets than on the {110} and {010} facets. A possible reason for the contrary conclusions is that the reaction selectivity on different facets is also affected by adsorption/desorption behaviours of reactant molecules and reaction intermediates on different facets [33] , [34] . A semiconductor with 1- D nanostructure and different crystal orientations has been proposed to lead to more efficient separation of electrons and holes with respect to the bulk material to explain the increased solar energy conversion efficiency [35] , [36] , [37] , [38] , [39] , though experimental evidence on the separation of electrons and holes on different crystal facets remains elusive. Here, we present experimental evidence for the separation of electrons and holes between the {010} and {110} crystal facets of the model semiconductor bismuth vanadate (BiVO 4 ). Facet-selective photo-deposition of metal ions, combined with promotion of water oxidation in photoelectrochemical and photocatalytic processes, clearly indicates the separation of electrons and holes to different facets. Meanwhile, various precursors of different metal ions as well as some distinct electron donors/acceptors were employed for the metal photo-deposition to rule out the adsorption effect. Selection of BiVO 4 as a model photocatalyst BiVO 4 , as a visible-light-responsive photocatalyst, has attracted increasing attention in photocatalytic [15] , [40] , [41] , [42] and photoelectrochemical [43] , [44] , [45] water oxidation. In addition, the BiVO 4 with large crystal size and controllable exposed facets can be easily prepared. Combined with advantages such as superior light absorbance, good photocatalytic activity, smooth exposed facets and non-toxic properties, BiVO 4 is chosen as an ideal model photocatalyst. A large single crystal of monoclinic BiVO 4 was prepared by the hydrothermal method [46] , [47] , and characterised by XRD patterns, UV–vis spectra and SEM images. The as-prepared BiVO 4 powder shows a smooth surface, regular decahedron shape, good crystallinity and characteristic visible-light absorption ( Supplementary Fig. S1 ). Facet-selective photo-deposition of metals/metal oxides The photo-depositions of metals on the surface of BiVO 4 were carried out using HAuCl 4 (H 2 PtCl 6 and AgNO 3 ) as precursors and water as a hole scavenger. SEM images ( Fig. 1a–d ) clearly show that the particles of Ag, Au and Pt (although with different particle sizes) are all solely deposited on the {010} facets. XPS spectra of Au 4f, Pt 4f and Ag 3d reveal that the deposited elements on the BiVO 4 are all in metallic form except that a small portion of incompletely reduced PtO species remained for the Pt/BiVO 4 sample ( Supplementary Fig. S2 ). Decrease of the metal valence with respect to the metal ion precursors indicates that the metal ions are photo-reduced on the {010} facets. Namely, the photogenerated electrons are readily available for the reduction reaction on the {010} facets. 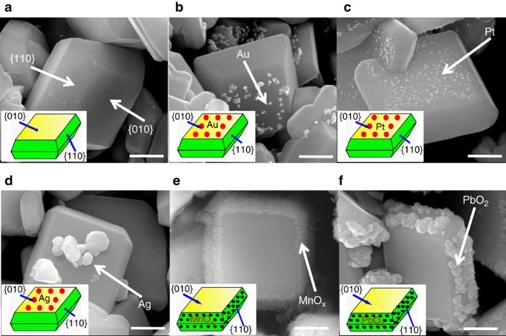Figure 1: SEM images of BiVO4with and without single metal/oxide deposited. (a) BiVO4; (b) Au/BiVO4; (c) Pt/BiVO4; (d) Ag/BiVO4; (e) MnOx/BiVO4and (f) PbO2/BiVO4. The contents of the deposited metals/metal oxides are all 5 wt%. Scale bar, 500 nm. The photo-reduction of metal ions (equation 1) accompanying the elimination of photogenerated holes by water oxidation (equation 2) can be described as follows: Figure 1: SEM images of BiVO 4 with and without single metal/oxide deposited. ( a ) BiVO 4 ; ( b ) Au/BiVO 4 ; ( c ) Pt/BiVO 4 ; ( d ) Ag/BiVO 4 ; ( e ) MnO x /BiVO 4 and ( f ) PbO 2 /BiVO 4 . The contents of the deposited metals/metal oxides are all 5 wt%. Scale bar, 500 nm. Full size image Photo-oxidation depositions of Mn 2+ or Pb 2+ ions on BiVO 4 were performed with IO 3 − as electron acceptors. Sponge-like manganese oxide deposits ( Fig. 1e ) and large lead oxide particles ( Fig. 1f ) are formed selectively on the {110} facets instead of the {010} facets. According to the binding energies of Pb 4f and Mn 2p in XPS ( Supplementary Fig. S3 ), the deposited lead and manganese species can be ascribed to PbO 2 and MnO x , respectively, where x is between 1.5 and 2.0 because the observed binding energies of manganese oxides are between those of Mn 2 O 3 and MnO 2 . High-resolution TEM images ( Supplementary Fig. S4 ) show that the planar spaces of 2.715 Å and 1.663 Å well match the (222) and (440) planes of cubic Mn 2 O 3 , and the planar space of 1.663 Å is in accordance with the (102) plane of hexagonal MnO 2 , further confirming the formation of MnO x . The formation of PbO 2 and MnO x oxides is an indication that the photo-oxidation selectively takes place on the {110} facets, that is, the photogenerated holes tend to migrate to the {110} facets for selective metal oxidation. The reactions can be summarised in equations (3) and (4): Following the selective photo-deposition of single metals and metal oxides, we further investigated the photo-deposition of dual precursors with simultaneous reduction and oxidation reactions. The as-prepared samples are denoted as Au/MnO x /BiVO 4 , Pt/MnO x /BiVO 4 , Ag/MnO x /BiVO 4 , Ag/PbO 2 /BiVO 4 , Au/PbO 2 /BiVO 4 and Pt/PbO 2 /BiVO 4 . It is interesting to note that the Au, Pt and Ag particles are still selectively photo-deposited on the {010} facets, while the MnO x and PbO 2 particles are loaded only on the {110} facets of BiVO 4 . This demonstrates that the facet-selective photo-deposition rules are also applied for the photo-deposition of dual components regardless of their combination order ( Fig. 2 ). The selective photo-deposition of the precursors is not obviously affected by the experimental conditions, supporting the fact that the {110} and {010} facets prefer the oxidation and reduction reaction, respectively. The mechanisms of the above-mentioned photo-depositions are schematically described in Fig. 3 , and the detailed experimental parameters are summarised in Supplementary Table S1 . All these results unambiguously reveal that the photogenerated electrons and holes tend to accumulate on the {010} and {110} facets, respectively, which results in the reduction and oxidation reactions taking place on the corresponding {010} and {110} facets. 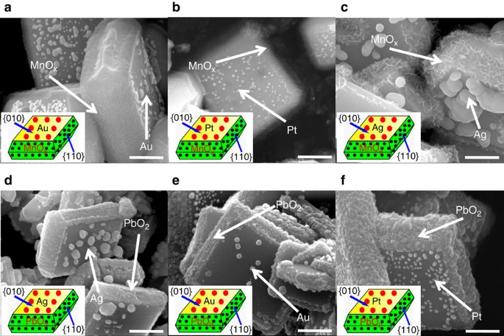Figure 2 SEM images of dual components photo-deposited on the surface of BiVO4. (a) Au/MnOx/BiVO4, (b) Pt/MnOx/BiVO4, (c) Ag/MnOx/BiVO4, (d) Ag/PbO2/BiVO4, (e) Au/PbO2/BiVO4and (f) Pt/PbO2/BiVO4. The contents of the deposited metals/metal oxides are all 5 wt %. Scale bar, 500 nm. Figure 2 SEM images of dual components photo-deposited on the surface of BiVO 4 . ( a ) Au/MnO x /BiVO 4 , ( b ) Pt/MnO x /BiVO 4 , ( c ) Ag/MnO x /BiVO 4 , ( d ) Ag/PbO 2 /BiVO 4 , ( e ) Au/PbO 2 /BiVO 4 and ( f ) Pt/PbO 2 /BiVO 4 . The contents of the deposited metals/metal oxides are all 5 wt %. Scale bar, 500 nm. 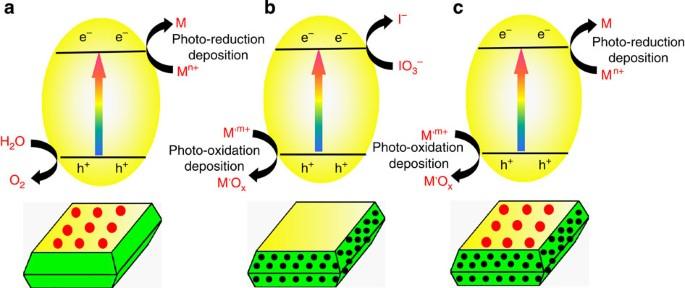Figure 3 Selective photo-deposition on BiVO4. (a) photo-reduction deposition of noble metals on the {010} facet, (b) photo-oxidation deposition of metal oxides on the {110} facet and (c) simultaneous photo-deposition of metal and metal oxides on the {010} and {110} facets, respectively. Full size image Figure 3 Selective photo-deposition on BiVO 4 . ( a ) photo-reduction deposition of noble metals on the {010} facet, ( b ) photo-oxidation deposition of metal oxides on the {110} facet and ( c ) simultaneous photo-deposition of metal and metal oxides on the {010} and {110} facets, respectively. Full size image Water oxidation by photoelectrochemical process In order to further illustrate the existence of the redox functional facets, the photoelectrochemical water oxidation of BiVO 4 with oxidation cocatalyst selectively deposited on different facets were examined. In this study, we prepared four typical photoanode electrodes denoted as BiVO 4 , MnO x (P.D. )/BiVO 4 , MnO x (imp)/BiVO 4 and IrO 2 (P.D. )/BiVO 4 , respectively. To achieve different deposition morphologies of the cocatalysts, the MnO x particles were deposited on the surface of BiVO 4 by two approaches. One is the selective photo-oxidation deposition introduced in this work (noted as MnO x (P.D. )/BiVO 4 ), and the other is the impregnation method that normally results in random dispersion (noted as MnO x (imp)/BiVO 4 ). Compared with the parent BiVO 4 electrode, the photoanode current in Fig. 4 is obviously increased when the oxidation cocatalyst MnO x is selectively deposited on the {110} facets, while the randomly dispersed MnO x on both {010} and {110} facets results in a slightly enhanced photocurrent. This demonstrates the photocurrent can be efficiently promoted only when the hole-trapping oxidation cocatalyst is selectively deposited on the {110} facets. On the other hand, the IrO 2 particles were firstly deposited by selective photo-deposition of metallic Ir particles on the {010} facets and subsequent calcination in air to convert the metallic iridium particles into IrO 2 . Decrease of photocurrent was observed for this sample with IrO 2 deposited on the {010} facets. This result indicates that if the cocatalysts deposited on the wrong facets, the photocurrent will be decreased. The typical SEM images ( Supplementary Fig. S5 ) of the deposited oxides confirmed that the photo-deposited MnO x and IrO 2 are selectively located on the {110} and {010} facets, respectively, while the MnO x (imp) particles are randomly dispersed on all facets. 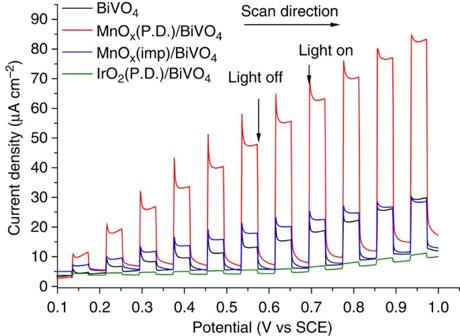Figure 4 Photochemical performances of four typical photoelectrodes. Black line: BiVO4; red line: MnOx(P.D.)/BiVO4; blue line: MnOx(imp)/BiVO4;green line: IrO2(P.D.)/BiVO4. P.D., photo-deposition, imp, impregnation. The MnOxnanoparticles on the MnOx(P.D.)/BiVO4are selectively deposited on the {110} facets, the MnOxparticles on the MnOx(imp)/BiVO4photoelectrodes are randomly dispersed on both {110} and {010} facets, and the IrO2nanoparticles on the IrO2(P.D.)/BiVO4electrode was deposited selectively on the {010} facets. The contents of the deposited cocatalysts are all 0.1 wt %. Reaction conditions: 0.5 M Na2SO4aqueous solution (pH=6.8). Light source, 300 W Xe lamp (λ≥420 nm), Scan rate: 10 mV s−1. Figure 4 Photochemical performances of four typical photoelectrodes . Black line: BiVO 4 ; red line: MnO x (P.D. )/BiVO 4 ; blue line: MnO x (imp)/BiVO 4; green line: IrO 2 (P.D. )/BiVO 4 . P.D., photo-deposition, imp, impregnation. The MnO x nanoparticles on the MnO x (P.D. )/BiVO 4 are selectively deposited on the {110} facets, the MnO x particles on the MnO x (imp)/BiVO 4 photoelectrodes are randomly dispersed on both {110} and {010} facets, and the IrO 2 nanoparticles on the IrO 2 (P.D. )/BiVO 4 electrode was deposited selectively on the {010} facets. The contents of the deposited cocatalysts are all 0.1 wt %. Reaction conditions: 0.5 M Na 2 SO 4 aqueous solution (pH=6.8). Light source, 300 W Xe lamp ( λ ≥420 nm), Scan rate: 10 mV s −1 . Full size image Water oxidation by photocatalysis Photocatalytic water oxidation using a powder photocatalyst was also evaluated for the BiVO 4 samples modified with reduction or/and oxidation cocatalysts. The cocatalysts were deposited by two methods: one is the facet-selective photo-deposition employed in this work to realise the selective deposition on a specific facet, the other is impregnation method normally resulting in random dispersion of deposited cocatalysts on all facets of BiVO 4 ( Supplementary Fig. S6 ). As shown in Fig. 5 , the photocatalytic oxygen evolution activity is strongly dependent on the species of cocatalyst and the deposition methods. The highest water oxidation activity is achieved for the Pt(P.D. )/MnO x (P.D. )/BiVO 4 sample with metallic platinum and MnO x particles selectively photo-deposited on the {010} and {110} facets, respectively. It should be pointed out that the contents of the deposited MnO x and Pt for photocatalytic water oxidation were all optimised to 0.1 wt% per ICP–AES analysis. The deposited metallic platinum on the {010} facets can collect electrons to reduce IO 3 − ions, and the MnO x particles photo-deposited selectively on the {110} facets can accumulate holes for water oxidation. Although sizes of the deposited platinum particles are similarly in the range of 10~30 nm for the cocatalysts located by both photo-deposition and impregnation methods, the promotion effect of cocatalysts deposited by impregnation method is not as evident as that by the photo-deposition. This result indicates that when the reduction/oxidation cocatalysts are selectively deposited on the corresponding reduction/oxidation reaction facets, namely when the cocatalysts are on the right facets of BiVO 4 , the photocatalytic performance can be most greatly enhanced. 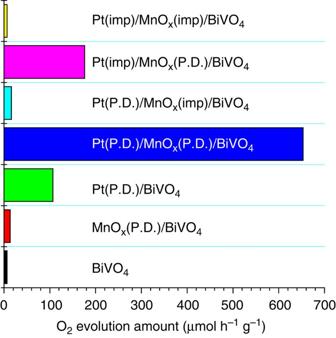Figure 5 Photocatalytic water oxidation performance of BiVO4. Reaction conditions: 150 ml 0.02 M NaIO3aqueous solution, 300 W Xe lamp (λ≥420 nm), top irradiation, reaction time: 1 h. (imp, impregnation method; P.D., photo-deposition method; the contents of the deposited cocatalysts are all 0.1 wt%). Figure 5 Photocatalytic water oxidation performance of BiVO 4 . Reaction conditions: 150 ml 0.02 M NaIO 3 aqueous solution, 300 W Xe lamp ( λ ≥420 nm), top irradiation, reaction time: 1 h. (imp, impregnation method; P.D., photo-deposition method; the contents of the deposited cocatalysts are all 0.1 wt%). Full size image Photocatalytic reactions can usually be used to explore the reduction and oxidation sites of photocatalysts, because the photogenerated electrons just work for the photo-reduction reaction, while the photogenerated holes are only available for the photo-oxidation [48] . It is reasonable to deduce that if a crystal facet selectively accumulates electrons or holes, the facet will just work for reduction or oxidation separately. As a result, metals/oxides can be selectively deposited on the specific facets via photo-reduction or photo-oxidation reactions. On the other hand, if a certain crystal facet of a semiconductor equally traps both photogenerated electrons and holes, the photo-reduction and photo-oxidation reactions could proceed on the same crystal facet. In this case, the selective photo-deposition of metal ions on the facets would also occur due to the existence of two possibilities: one is the accumulation of electrons or holes on the facet, the other is the selective adsorption of the reactants on the given facet [34] . The possibility for preferential adsorption of anions or selective adsorption of metal ions, leading to selective photo-deposition, can be ruled out in this work because of the following experimental facts. On the one hand, various metal precursors (AgNO 3 , HAuCl 4 , H 2 PtCl 6 , Pb(NO 3 ) 2 , MnSO 4 ) with different anionic species such as Cl − , NO 3 − and SO 4 2− are employed, but the selective photo-deposition of metals and oxides are not changed. For example, the deposition of noble metals Au, Pt and Ag from precursors with distinct anions always selectively proceeded on the {010} facets of BiVO 4 photocatalyst. On the contrary, the deposition of Ag and PbO 2 on the {010} and {110} facets, respectively, are observed when the precursors with the same NO 3 − anions are applied. Moreover, the manganese ions are similarly deposited on the {110} facets ( Supplementary Fig. S7 ) even though the precursors with distinct anions, such as Cl − , SO 4 2− and NO 3 − and so on, are applied. On the other hand, the isoelectric point of BiVO 4 was measured to be about 3.5, close to the values reported in the literature [49] , [50] , which is slightly lower than the pH values of the photo-deposition solutions ( Supplementary Table S1 ), indicating that the surfaces of BiVO 4 are negatively charged during the photo-deposition. As a consequence, the adsorption of AuCl 4 − or PtCl 6 2− anions on the surface of BiVO 4 should be less favourable than that of Ag + , Pb 2+ or Mn 2+ cations in consideration of adsorption competition of ions with the same charge. However, the gold and platinum complex anions (AuCl 4 − , PtCl 6 2− ) and silver cations (Ag + ) are all photo-reduced selectively on the {010} facets, while both the lead and manganese cations are photo-oxidised on the {110} facets. In addition, we also attempted to deposit noble Au, Pt and Ag by employing methanol instead of water as hole scavengers, and found that all of these metals are selectively deposited on the {010} facets of BiVO 4 ( Supplementary Fig. S8 ). Therefore, the influence of adsorption on the selective photo-deposition behaviours caused by the pH environment, absorption of special ions and organic sacrificial reagent like methanol can also be ruled out. Exclusion of the adsorption effect originating from the precursor ions and preparative environments renders us to reasonably ascribe the facet-selective photo-deposition of metals and oxides to the accumulation of electrons and holes on the {010} and {110} facets of BiVO 4 , respectively, which correspondingly function as reduction and oxidation facets. It is reasonable to deduce that the accumulation of electrons and holes originates from charge separation on different facets. The origin of the charge separation on the {010} and {110} crystal facets of TiO 2 has been already estimated by theoretical calculation [19] . Similarly, we also evaluated the energy levels of {010} and {110} facets of BiVO 4 by DFT calculation method. A slight difference in energy of the valance and conduction band between {010} and {110} facets ( Supplementary Fig. S9 ) suggests that the electron transfer from {110} to {010} facets is feasible thermodynamically, leading to the accumulation of electrons and holes separately on the {010} and {110} facets. It is worth noting that the band bending of each facet may be distinct due to their different surface electronic structures, as should be another factor affecting the spatial charge separation. To further confirm the efficient charge separation on different crystal facets, the influence of temperature on the facet-selective photo-deposition was also examined ( Supplementary Fig. S10 ). The morphology of the facet selectively deposited Au and MnO x is independent of the temperature in the experimental conditions (<100 °C), except that the particle size of the deposited metals is slightly varied with increasing deposition temperature. The temperature-independent facet-selective metal deposition also indicates that the facet-selective deposition is not due to the selective adsorption effect which is usually temperature dependent. The separation of the photogenerated electrons and holes on the {010} and {110} facets of BiVO 4 is further supported by our photoelectrochemical or photocatalystic water oxidation reaction. It has been known that if the oxidation cocatalyst is deposited on the oxidation sites of the photoelectrode, the photoanode currents can be increased because hole trapping on the oxidation cocatalyst can lead to better charge separation [51] , [52] , [53] , [54] , [55] . Indeed, our photoelectrochemical measurements show that the photoanode current was remarkably enhanced when the MnO x was selectively photo-deposited on the hole-concentrated {110} facets of BiVO 4 ( Fig. 3 ). In contrast, when the oxidation cocatalyst IrO 2 was controllably deposited on the electron-accumulated {010} facet, the performance of water oxidation is inhibited. Similarly, only when reduction cocatalyst Pt and oxidation cocatalyst MnO x are selectively photo-deposited on the {010} and {110} facets of BiVO 4 , the photocatalytic activity of water oxidation can be most greatly enhanced ( Fig. 4 ). Based on these observations, we conclude that the photogenerated electrons and holes on the surface of BiVO 4 are accumulated on the {010} and {110} facets for reduction and oxidation reaction, respectively. In summary, taking BiVO 4 as a model semiconductor, we confirm the existence of oxidation and reduction facets, which are evidenced by facet-selective photo-deposition of metals and oxides, and promotion of photocatalytic or photoelectrochemical water oxidation reaction by controllable deposition of the oxidation/reduction cocatalysts on the corresponding oxidation/reduction facets. The observation of the functional facets of the BiVO 4 crystal reveals spatial separation of the photogenerated electrons and holes between {010} and {110} facets of BiVO 4 , which are mainly owing to the difference of energy levels of these facets. Our results also show the importance of the cocatalysts loading on the right crystal facets for efficient photocatalytic water splitting. The findings of functional redox facets, selective deposition of redox cocatalysts on the different facets of a single crystal, and efficient charge separation between different facets should be promising and intriguing for understanding the mechanism of photocatalytic reactions, and designing highly efficient solar energy conversion photocatalysts/devices. Facet-selective photo-deposition of metals and/or oxides BiVO 4 sample was synthesised by a hydrothermal procedure ( Supplementary Methods ). For the facet-selective photo-depositions, three ways containing single reduction, single oxidation as well as simultaneous reduction and oxidation were carried out at room temperature without pH value adjusted. Normally, 0.50 g BiVO 4 powder and a calculated amount of metal precursors (5 wt%) were mixed in 100 ml deionised water. The suspension was then irradiated by a 300-W Xe lamp ( λ ≥420 nm) under continuous stirring. After 5 h photo-deposition, the suspension was filtered, washed with deionised water for more than three times, and finally dried at 60 °C for overnight. For comparison, the simultaneous photo-deposition of gold and manganese was also carried out at 50 and 90 °C, respectively. The as-obtained powder was used for characterizations and/or activity tests. Preparation of photoelectrodes The BiVO 4 film electrodes were prepared by electrophoretic deposition on FTO substrate (1 × 2 cm 2 ) [47] , followed by drying in air and calcination at 573 K for 1 h. On the surface of the BiVO 4 electrode, different cocatalysts containing MnO x or IrO 2 were subsequently deposited. As for the MnO x deposition, two methods were employed for comparison. One is the {110} facet-selective photo-deposition method that was carried out in a Pyrex reactor in 0.01 M MnSO 4 solution containing 0.02 M NaIO 3 , and illuminated from the top using a 300-W Xe lamp. The other is the conventional impregnation method, that is, impregnation of Mn (NO 3 ) 2 solutions (0.01 M) on the BiVO 4 electrode followed by calcination under 573 K for 1 h. The as-prepared electrodes are denoted as MnO x (P.D. )/BiVO 4 and MnO x (imp)/BiVO 4 , respectively. The IrO 2 (P.D. )/BiVO 4 electrode was prepared by selective photo-deposition of metallic iridium on the {010} facet of BiVO 4 from 1 mM Na 2 IrCl 6 solution, which was transferred into IrO 2 by calcination in air at 573 K for 1 h. Water oxidation by photoelectrochemical process The Photoelectrochemical performances of the photoanodes were measured in a three-electrode setup, where Pt electrode and saturated mercury electrode were employed as counter and reference electrode, respectively. Electrolyte was 0.5 M Na 2 SO 4 (pH=6.8) solution. For linear sweep voltammetry, the potential was swept with scan rate of 10 mV s −1 . A shutter was used to record both the dark and photocurrent during a single scan. A 300-W Xe lamp (Ushio-CERMAXLX300) and optical cutoff filter (Kenko, L-42; λ ≥420 nm) was used as light source. The contents of the deposited cocatalysts are all 0.1 wt% regardless of the methods, which were confirmed by ICP–AES analysis. Water oxidation by photocatalysis The photocatalytic O 2 evolution reactions were carried out in a closed gas circulation and evacuation system using a 300-W Xe lamp (Ushio-CERMAXLX300) and optical cutoff filter (Kenko, L-42; λ ≥420 nm). Normally, 0.15 g photocatalyst was dispersed in 150 ml 0.02 M NaIO 3 aqueous solution in a Pyrex reaction cell. Before irradiation, the reaction system was thoroughly degassed by evacuation in order to drive off the air inside. The amount of evolved O 2 was determined by an online gas chromatograph (Agilent, GC-7890, TCD, Ar carrier). The rate of O 2 evolution in the initial 1 h was recorded for comparison. The contents of the deposited cocatalysts are all 0.1 wt% regardless of the methods, which were confirmed by ICP–AES analysis. How to cite this article: Li, R. et al . Spatial Separation of Photogenerated Electrons and Holes among {010} and {110} Crystal Facets of BiVO 4 . Nat. Commun. 4:1432 doi: 10.1038/ncomms2401 (2013).